Correspondence: Oncogenic MYC persistently upregulates the molecular clock component REV-ERBα 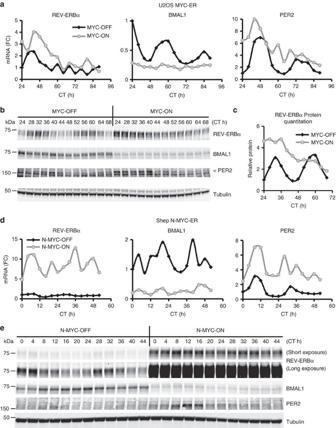Figure 1: MYC and N-MYC induce persistent elevation of REV-ERBα mRNA and protein. (a,b) U2OS BMAL1::Luc cells expressing MYC-ER were cultured±4OHT (with ethanol serving as a loading control for all experiments) for 24 h, then changed to ‘lumicycle’ media (see Methods)±4OHT and+0.1 μM dexamethasone. (a) mRNA was collected at the indicated time points after synchronization, and endogenous REV-ERBα (NR1D1), BMAL1 (ARNTL), and PER2 were determined by RT-PCR, normalized to β2M. mRNA (FC)=fold change. (b) Lysates were collected at the indicated time points after synchronization and processed for protein expression of REV-ERBα, BMAL1, and PER2 (indicated by <). Tubulin serves as a loading control. Portions of a and b were previously published1, but instead labelled as 0–48 h. (c) REV-ERBα protein from (b) was quantitated using Image Studio software (Licor, Lincoln, NE, USA), normalized to the relevant Tubulin and plotted over time. (d,e) SHEP N-MYC-ER expressing cells10were cultured±4OHT for 24 h, then 0.1 μM dexamethasone was added. (d) mRNA was collected at the indicated time points after synchronization, and endogenous REV-ERBα (NR1D1), BMAL1 (ARNTL) and PER2, were determined by RT-PCR, normalized to β2M. (e) Lysates were collected at the indicated time points after synchronization and processed for protein expression of REV-ERBα (‘short’ and ‘long’ indicate exposure time), BMAL1 and PER2. Tubulin serves as a loading control. For all panels, CT (cell time) indicate time of collection after synchronization. For immunoblots, molecular weights are noted in kDa. Portions ofa–cwere previously published1and are reprinted with permission from Elsevier. 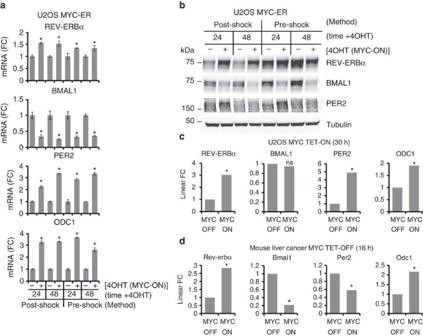Figure 2: REV-ERBα mRNA is induced by MYC regardless of synchronization method and in multiple cell line and tumor models. (a,b) MYC was induced in U2OS MYC-ER cells that were synchronized with dexamethasone in two different schemes. ‘Post-Shock’1: as inFig. 1, cells were treated±4 OHT (with ethanol serving as a loading control for all experiments) for 24 h. The ‘24’ h sample was collected, then 0.1 μM dexamethasone was added to media and the ‘48’ h sample was collected 24 h later. ‘Pre-Shock’2: 1 μM dexamethasone was added for 20 min, then cells were washed once in PBS and fresh media was added±4OHT. Cells were collected at the indicated times after media change. (a) mRNA was collected at the indicated times, and endogenous REV-ERBα (NR1D1), BMAL1 (ARNTL),PER2, andODC1were determined by RT-PCR, normalized to β2M. mRNA (FC)=fold change. Data are averages of biological triplicates with error bars representing s.d., and *P<0.05 by Student’st-test of 4 OHT (MYC-ON) samples relative to ethanol (MYC-OFF) samples at each time point. (b) Samples from (a) were processed for protein expression of REV-ERBα, BMAL1 and PER2. Tubulin serves as a loading control. Molecular weights are noted in kDa. (c) Previously published RNA-Seq data13from U2OS cells expressing exogenous MYC under the control of a TET-ON system and treated±1 μg ml−1doxycycline for 30 h. REV-ERBα (NR1D1), BMAL1 (ARNTL),PER2andODC1were determined. Data are presented as linear fold change (FC) and represent biological triplicates, and *P<0.05 of MYC-ON samples relative to MYC-OFF samples as previously described13; NS, not significant. (d) Previously published RNA-seq data14from liver tumors driven by a MYC-TET-OFF system. Mice were fed water or doxycycline for 16 h to turn off MYC. Rev-erbα (Nr1d1), Bmal1 (Arntl),Per2andOdc1were determined. Data are presented as linear FC and represent biological duplicates, and *P<0.05 of MYC-ON samples relative to MYC-OFF samples as previously described14. Cell culture U2OS BMAL1::Luc MYC-ER (oestrogen receptor Tamoxifen Mutant) was derived by stable expression of pBabe-Zeo MYC-ER in U2OS BMAL1::Luc cells [12] , and subsequent selection and culture with 100 μg ml −1 Zeocin (Life Technologies, Grand Island, NY, USA) [1] . Murine hepatocellular carcinoma cell line (mHCC) 3–4, a primary culture tumour cell line, was derived by ring cloning of a liver tumour from the LAP-tTA/tet-OFF cMYC conditional transgenic mouse liver cancer model [6] , [7] . U2OS, mHCC 3–4, Shep N-MYC-ER [10] and SKNAS N-MYC-ER [11] were cultured in Dulbecco’s Modified Eagle’s Medium (DMEM, Mediatech, Manassas, VA, USA) containing glucose at 25 mM and glutamine at 4 mM. Media was supplemented with 10% fetal bovine serum (FBS, HyClone, Logan, UT, USA or Life Technologies) and 1X Penicillin/Streptomycin (Mediatech). mHCC cells were additionally supplemented with 2 mM glutamine (Mediatech), 1 mM sodium pyruvate (Mediatech) and 1X MEM non-essential amino acids (Life Technologies). P493-6 cells [5] , [9] were cultured in RPMI-1640 medium (Mediatech) with 10% FBS (HyClone or Life Technologies) and 1X Penicillin/Streptomycin (Mediatech). All cell culture was conducted in a 5% CO 2 humidified atmosphere. For collecting cells, cells were washed one time in PBS (Life Technologies), removed from the plate with Trypsin-EDTA 0.25% (Life Technologies), suspended in media, spun down and then processed as indicated. To activate MYC-ER or N-MYC-ER, U2OS, SHEP and SKNAS cells were treated with 500 nM 4-hydroxytamoxifen (Sigma, St Louis, MO, USA) or ethanol control. To suppress MYC expression, mHCC 3-4 cells were treated with 20 ng ml −1 tetracycline (Sigma) or media control for 24 h, and P493-6 cells were treated with 100 ng ml −1 tetracycline or media control for 24 h. To induce intermediate MYC expression (Int. MYC), P493-6 cells were treated+100 ng ml −1 tetracycline and 1 μM β-estradiol (Sigma) for 1 week, then cultured in β-estradiol±tetracycline for experiments. U2OS BMAL1::Luc parental and MYC-ER were authenticated using the Cell Check 16 service (IDEXX Bioresearch, Columbia, MO, USA) with cell pellets that had been frozen. Authentication confirmed that the cells were free of interspecies contamination and genetically identical to a published U2OS profile using a detailed 16-STR (short tandem repeat) screen. U2OS BMAL1::Luc MYC-ER, mHCC 3-4 and p493-6 cells were tested for mycoplasma and found to be negative. SHEP N-MYC-ER and SKNAS N-MYC-ER were not tested. Real-time PCR and primers mRNA was extracted using the RNEasy Plus Mini Kit (Qiagen, Gaithersburg, MD, USA) following manufacturer’s instruction and then reverse-transcribed to cDNA by using TaqMan Reverse Transcription Reagents (Life Technologies). cDNA was used as template for quantitative real-time PCR (RT-PCR) with specific human or mouse primers. All RT-PCRs in this work were performed using the ViiA 7 Real-time PCR system (Life Technologies). Relative mRNA expression levels were normalized to β2M and analysed using comparative delta-delta CT method. RT-PCR primers and sources of these primers are listed in Supplementary Table 3 , in the Supplementary Information section. Circadian time-series sample collection All circadian time-series experiments were performed in the media described above, with U2OS, SHEP, SKNAS and mHCC 3–4 cells synchronized by addition of 0.1 μM dexamethasone (Sigma) to growth media before start of collection. As an exception, for Fig. 1a–c , U2OS MYC-ER cells were switched to ‘lumicycle media’ containing dexamethasone at the start of the experiment: phenol red-free DMEM (Sigma) containing 5% FBS (Hyclone or Life Technologies), 25 mM D-glucose (Sigma), 35 mg l −1 sodium bicarbonate (Thermo Fisher, Grand Island, NY), 10 mM HEPES (Thermo Fisher) and Pen/Strep (Mediatech). P493-6 cells were ‘serum shocked’ in 50% FBS+growth media for 2 h, then replated in normal growth media at the start of time-series collection [8] . All time-series experiments were performed as a ‘split-timecourse’: 24 h before to the start of the experiment, half the cells were synchronized with 0.1 μM dexamethasone (dex, Sigma), and at the start of the experiment, the other half of the cells were synchronized with dexamethasone. At each time point, two plates were collected representing 0 and 24 h +dex, 4 and 28 and so on, to arrive at a 52 h time series. For all time-series experiments, CT denotes circadian time. mRNA and protein were processed and analysed as described above. Comparison of synchronization methods To compare synchronization methods between labs, we employed ‘Pre-Shock’ [1] , [12] : U2OS MYC-ER cells were first treated±4OHT for 24 h, then some cells were collected for protein and mRNA 24 h later, and others were synchronized with 0.1 μM dexamethasone and collected at 48 h±4OHT. For the method employed by Shostak et al . [2] (‘Post-Shock’), we treated U2OS MYC-ER cells with 1 μM dexamethasone for 20 min, washed once in PBS, then cultured the cells in normal medium±4OHT. Cells were collected for mRNA and protein 24 and 48 h later. Immunoblots and immunoblot quantitation Cells were lysed for at least 20 min in M-PER Mammalian Protein Extraction Reagent (Thermo Fisher) supplemented with protease inhibitor cocktail (BD Biosciences, San Jose, CA, or Promega, Madison, WI, USA) and phosphatase inhibitors II and III (Sigma). Lysates were centrifuged at 16,000 g for 10 min at 4 °C, and supernatants were saved for quantitation and analysis. Protein content was quantified using the Bio-Rad DC assay kit (Bio-Rad, Hercules, CA, USA), with BSA serving as a reference (Thermo Fisher). Proteins were separated by SDS-PAGE using Criterion pre-cast gradient gels (Bio-Rad). Molecular weight was determined by comparison with Precision-Plus Dual Xtra protein standards (Bio-Rad). Primary antibodies used include: rabbit anti-REV-ERBα (1:1,000, #13418S, Cell Signaling, Danvers, MA, USA); rabbit anti-BMAL1 (1:1,000, #14020S, Cell Signaling); rabbit anti-PER2 (1:1,000, #20359-1-AP, Proteintech, Chicago, IL, USA); rabbit anti-c-MYC (1:10,000, #ab32072, Abcam, Cambridge, MA, USA); rabbit anti-CRY1 (1:1,000, #ab104736, Abcam); and mouse anti-α-Tubulin (1:10,000, #CP06, EMD Millipore, Billerica, MA, USA). Secondary antibodies used include: Alexa-Flour 680 goat anti-rabbit IgG (1:8,000, #A21109, Life Technologies, Grand Island, NY); Alexa-Flour 790 goat anti-mouse IgG (1:8,000, #A11357, Life Technologies); and IRDye 800CW Goat Anti-Mouse IgG (1:10,000, #926-32210, Licor, Lincoln, NE). Immunoblots were imaged with the Odyssey CLx infrared imaging system (Licor) and uniformly contrasted. Immunoblots were quantitated using the Licor Image Studio software. For each band, median background intensity with a 3 pixel border width was automatically subtracted. Each REV-ERBα band value was normalized against the applicable Tubulin band, and then all the quantitated bands were further normalized by arbitrarily setting the MYC-OFF CT 24 value to 1 and dividing all the others by this value. Raw, uncropped images of all immunoblots are presented in Supplementary Figs 4–8 , along with molecular weight markers for each blot. Statistical analysis For all single-time point mRNA expression data with biological replicates, error bars represent s.d., and * P <0.05 by Student’s t -test from three experiments. For publically available data, * P <0.05 as previously described [13] , [14] . Data availability For U2OS MYC TET-ON RNA-Seq, publically available data was used from Walz et al . [13] (GEO accession # GSE44672, sample ID # GSM1231609). Data were supplied as log fold-change and were linearized for this work. For mouse hepatocellular carcinoma MYC TET-OFF samples, publically available data was used from Kress et al . [14] , supplied in a Supplementary Figure to their work. Data were supplied as log fold-change and were linearized for this work. All other relevant data are available from the authors. How to cite this article: Altman, B. J. et al . Correspondence: Oncogenic MYC persistently upregulates the molecular clock component REV-ERBα. Nat. Commun. 8, 14862 doi: 10.1038/ncomms14862 (2017). Publisher’s note : Springer Nature remains neutral with regard to jurisdictional claims in published maps and institutional affiliations.